Adipocyte YTH N(6)-methyladenosine RNA-binding protein 1 protects against obesity by promoting white adipose tissue beiging in male mice Obesity, one of the most serious public health issues, is caused by the imbalance of energy intake and energy expenditure. N(6)-methyladenosine (m 6 A) RNA modification has been recently identified as a key regulator of obesity, while the detailed mechanism is elusive. Here, we find that YTH RNA binding protein 1 (YTHDF1), an m 6 A reader, acts as an essential regulator of white adipose tissue metabolism. The expression of YTHDF1 decreases in adipose tissue of male mice fed a high-fat diet. Adipocyte-specific Ythdf1 deficiency exacerbates obesity-induced metabolic defects and inhibits beiging of inguinal white adipose tissue (iWAT) in male mice. By contrast, male mice with WAT-specific YTHDF1 overexpression are resistant to obesity and shows promotion of beiging. Mechanistically, YTHDF1 regulates the translation of diverse m 6 A-modified mRNAs. In particular, YTHDF1 facilitates the translation of bone morphogenetic protein 8b ( Bmp8b ) in an m 6 A-dependent manner to induce the beiging process. Here, we show that YTHDF1 may be an potential therapeutic target for the management of obesity-associated diseases. Adipose tissue is traditionally categorized into white adipose tissue (WAT) and brown adipose tissue (BAT), depending on its morphology and function [1] . WAT possesses unilocular, large lipid droplets and is involved in lipid storage. Excessive lipid storage in WAT results in obesity and related metabolic disorders, including insulin resistance, hepatic steatosis, diabetes, and cardiovascular disease [2] , [3] . By contrast, BAT possesses multilocular, small lipid droplets and a large number of mitochondria, in which uncoupling protein 1 (UCP1) is expressed, specializing in energy production in the form of heat [4] . Emerging evidence has identified a third type of adipose tissue, termed “beige” adipose tissue, which can be induced from WAT in cases of cold exposure, exercise, diet, and various activators [5] , [6] . Beige adipose tissue has unique origins and molecular characteristics compared with classic BAT [7] . Activation of thermogenesis in brown or beige adipose tissues increases systemic energy expenditure and alleviates obesity-associated metabolic diseases [8] , [9] . Thus, a deeper understanding of the mechanisms regulating energy storage and expenditure may lead to the development of therapeutic strategies that improve metabolic health. N(6)-methyladenosine (m 6 A), the most abundant internal modification on mRNA, is catalyzed by the RNA methyltransferase complex methyltransferase-like (METTL) 3/METTL14/WT1-associated protein [10] , [11] , [12] . As a reversable modification, m 6 A methylation can be removed by AlkB homolog 5 or fat mass and obesity-associated protein (FTO) [13] , [14] . The YTH domain-containing ‘reader’ proteins, bind m 6 A and differentially regulate mRNA metabolism, including mRNA splicing, maturation, degradation, and translation. YTHDF1 enhances the translation of m 6 A-modified mRNAs, while YTHDF2 promotes the degradation of m 6 A-modified mRNAs [15] , [16] . YTHDF3 was reported to regulate both mRNA translation and degradation [17] . Recent studies have highlighted an essential role of m 6 A modification in adipocytes metabolism. Single-nucleotide polymorphisms in FTO are closely related to the occurrence of obesity [18] , [19] , and knockout of Fto decreases HFD-induced obesity [20] . Coordinately, FTO inhibitors can increase thermogenesis, improve glucose tolerance, and ultimately inhibit obesity [21] . Moreover, METTL3 is essential for controlling postnatal development and energy homeostasis in BAT [22] . Because the fates of methylated mRNAs, ranging from degradation to translation, are determined by their reader proteins [15] , [16] , [23] , [24] , deciphering the functions of m 6 A reader proteins may help elucidate the mechanisms of m 6 A function in adipocyte metabolism. In this work, we assessed the role of YTHDF1 in adipose tissue using WAT-specific Ythdf1 -knockout male mice and adeno-associated virus [25] -mediated Ythdf1 overexpression. We demonstrated that YTHDF1 promotes mRNA translation to induce WAT beiging and alleviate obesity. Our results highlighted an important role of YTHDF1 in preventing obesity and provided potential targets for the treatment of obesity-associated metabolic diseases. Adipose YTHDF1 expression is reduced in obesity Dysregulated m 6 A modification results in obesity in both mice and human beings [18] , [19] . To investigate the functions of “reader” proteins in this process, we detected the expression of YTH proteins (YTHDF1/2/3) in mice fed a standard chow diet (CD) or obese mice induced by a high fat diet (HFD). We observed a dramatic increase in body weight, iWAT weight, eWAT weight and BAT weight, indicating the successful induction of obesity (Supplementary Fig. 1A ). Interestingly, YTHDF1 was dramatically downregulated in inguinal WAT (iWAT) in obese mice compared with that in control mice (Fig. 1a, c , Supplementary Fig. 1B, C ). The expression of YTHDF2/3 did not change in both iWAT and BAT of HFD-induced mice (Fig. 1a–d , Supplementary Fig. 1B–E ). Notably, HFD-fed mice exhibited lower expression of thermogenic genes (e.g., Ucp1 , Ppargc1a , Cidea , Pparg , Adrb3 , and Cox8b ) in iWAT, implying impaired thermogenesis (Fig. 1c ). Importantly, the published sequencing data revealed decreased YTHDF1 mRNA expression in WAT of individuals with obesity compared with that in nonobese individuals (Fig. 1e ). The negative correlation of YTHDF1 expression in WAT with obesity implies a role of this protein in adipose tissue metabolism. Fig. 1: Adipose YTHDF1 expression is reduced in obesity. a , b Immunoblot analysis of YTH family proteins in iWAT a and BAT b of mice fed with CD or HFD for 12 weeks. c, d mRNA levels of Yth family genes and thermogenesis-related genes in iWAT c and BAT d of CD- and HFD-fed mice. Data were presented as mean ± SEM ( n = 10). ns, not significant, * P < 0.05, ** P < 0.01, *** P < 0.001, two-sided t-test. e Expression of YTHDF1 in human white adipose tissues from GSE156906 ( n Lean = 14, n Obesity = 27, two-sided t-test), GSE162653 ( n = 10, two-sided t-test), and GSE110729 ( n Lean = 15, n Obesity = 13, F-test). Source data are provided as a Source Data file. Full size image Adipocyte-specific knockout of Ythdf1 predisposes mice to HFD-induced obesity To study the function of YTHDF1 in adipose tissue, we generated adipocyte-conditional Ythdf1 -knockout mice ( Ythdf1 cKO mice, termed Y1 cKO or cKO), which were produced by crossing Ythdf1 flox/flox mice ( Ythdf1 CTL mice, termed Y1 CTL or CTL) with Adipoq-Cre transgenic mice (Supplementary Fig. 2A , Fig. 2a ). Knockout of Ythdf1 did not affect the expression of YTHDF2/3 in iWAT and BAT (Supplementary Fig. 2B, C ). CD-fed Ythdf1 cKO mice and Ythdf1 CTL littermates showed similar weight gain and similar iWAT, BAT, and eWAT weights (Supplementary Fig. 2D, E ). Consistent with these results, there were no difference in triglyceride (TG), total cholesterol (CHO), or low-density lipoprotein (LDL) levels between Ythdf1 CTL and Ythdf1 cKO mice after CD feeding (Supplementary Fig. 2F ). Analyses of intraperitoneal glucose tolerance and insulin resistance, as measured using glucose tolerance tests (GTTs) and insulin tolerance tests [26] , showed no significant difference between CD-fed Ythdf1 CTL and Ythdf1 cKO mice (Supplementary Fig. 2G, H ). Fig. 2: Adipocyte-specific knockout of Ythdf1 predisposes mice to HFD-induced obesity. a Immunoblotting of adipose tissues from Y1 CTL and Y1 cKO mice. b Schematic of the mouse treatment regimen. c – n The Y1 CTL and Y1 cKO littermates were fed with HFD. c Daily food intake by Y1 CTL and Y1 cKO mice. d Gross view of Y1 CTL and Y1 cKO mice. Scale bar, 0.5 cm. e Body weights of Y1 CTL and Y1 cKO mice. f Gross view and weights of iWAT, eWAT, and BAT from Y1 CTL and Y1 cKO mice. Scale bar, 0.5 cm. g H&E staining of iWAT eWAT, and BAT from Y1 CTL and Y1 cKO mice. Scale bar, 50 μm. The red line indicated the average size. No adjustments. h – j O 2 consumption h , CO 2 generation i , and energy heat generation j of Y1 CTL and Y1 cKO mice. White and gray areas in the graphs indicate day and night, respectively. k Rectal temperature in Y1 CTL and Y1 cKO mice. l Serum concentrations of TG, CHO, LDL, and HDL in Y1 CTL and Y1 cKO mice fed with HFD. m , n glucose tolerance m and Insulin tolerance n fed with HFD. Data in c , e – n were presented as mean ± SEM ( n = 4 biologically independent mice). ns, not significant, * P < 0.05, ** P < 0.01, **** P < 0.0001, two-sided t-test. Source data are provided as a Source Data file. Full size image To clarify the function of YTHDF1 in obesity, Ythdf1 CTL and Ythdf1 cKO mice were fed an HFD starting at 10 weeks of age to induce obesity (Fig. 2b ). Although CD-fed Ythdf1 cKO mice and Ythdf1 CTL littermates showed similar weight gain (Fig. 2e ), HFD-fed Ythdf1 cKO mice showed significantly higher body weights compared with Ythdf1 CTL littermates, despite comparable food intake (Fig. 2c–e ). Examination of dissected fat tissues confirmed that epididymal and inguinal but not brown fat pads were larger in Ythdf1 cKO mice (Fig. 2f ). Moreover, hematoxylin and eosin (H&E) analysis revealed that the WAT in Ythdf1 cKO mice showed enhancement of obesity-related features, including larger unilocular lipid droplets (Fig. 2g ). Taken together, these data suggested that Ythdf1 cKO mice were more prone to HFD-induced obesity. Adipocyte-specific knockout of Ythdf1 aggravates obesity-induced metabolic disorders The observed increase in body weight after HFD feeding, independent of food intake, suggested increased energy storage and reduced thermogenesis by Ythdf1 cKO mice. Indeed, metabolic cage experiments demonstrated that deletion of Ythdf1 inhibited oxygen consumption, carbon dioxide generation, and energy heat generation during dark cycles (Fig. 2h–j ). The core temperature was significantly reduced in Ythdf1 cKO mice (Fig. 2k ). HFD feeding can elevate circulating levels of TG, CHO, and LDL [27] . We observed a further increase in these parameters in HFD-fed Ythdf1 cKO mice (Fig. 2l ). Notably, GTTs and ITTs showed that Ythdf1 cKO mice fed an HFD developed glucose intolerance and insulin resistance (Fig. 2m, n ). Collectively, our data demonstrated that adipocyte-specific knockout of Ythdf1 aggravated the detrimental effects of obesity. Furthermore, we fed the Ythdf1 CTL and Ytdhf1 cKO mice HFD under thermoneutral conditions. Deletion of Ythdf1 exacerbated obesity, reduced rectal temperature, and downregulated the thermogenic genes (Supplementary Fig. 3A–E ). Metabolic cage experiments showed that deletion of Ythdf1 inhibited oxygen consumption, carbon dioxide generation, and energy heat generation during both light and dark cycles (Supplementary Fig. 3F–H ). These data implied that the metabolic changes in Ythdf1 cKO mice might be caused by impaired thermogenesis of iWAT. Adipocyte-specific knockout of Ythdf1 inhibits the beiging of WAT Studies have demonstrated that beige adipose tissue plays active roles in lipid metabolism and has potential therapeutic relevance for weight loss [8] , [28] . Beiging is induced by chronic exposure to external cues, such as cold treatment or adrenergic stimulation [5] , [6] . To investigate whether YTHDF1 modulates the functions of beige adipose tissues, we induced the beiging process. YTHDF1, but not YTHDF2/3, was upregulated in cold-treated iWAT (Fig. 3a and Supplementary Fig. 4A, B ). β3-Adrenergic receptor (AR) is the main signaling protein involved in the beiging process. Intraperitoneal administration of the β3-AR agonist CL-316,243 (CL) resulted in the upregulation of YTHDF1 (Fig. 3b ). Histological and immunohistochemical analyses showed that the lipid droplets were larger in Ythdf1 cKO mice than that in Ythdf1 CTL mice after cold stimulation (Fig. 3c ). UCP1 expression was also dramatically downregulated in iWAT of Ythdf1 cKO mice (Fig. 3d ). Overexpression of YTHDF2/3 could not rescue the phenotype of Ythdf1 cKO (Supplementary Fig. 4C, D ), implying differential roles of YTHDF1/2/3 in adipose tissue. Interestingly, UCP1 in BAT was unchanged in Ythdf1 cKO mice after cold stimulation (Fig. 3e ). Other thermogenesis- and lipolysis-related genes were both downregulated in iWAT rather than BAT (Fig. 3f, g and Supplementary Fig. 4E, F ), suggesting that YTHDF1 may have a major role in WAT rather than BAT. Consistently, the rectal temperatures of Ythdf1 cKO mice remained lower after cold exposure (Fig. 3h ). The primary preadipocytes were further isolated from Ythdf1 CTL and Ythdf1 cKO mice and the thermogenic program was determined. Deletion of Ythdf1 dramatically reduced the O 2 consumption rate (OCR) in primary preadipocytes (Fig. 3i ). Fig. 3: Adipocyte-specific knockout of Ythdf1 inhibits beiging of iWAT. a Immunoblot analysis of YTH family proteins expression in iWAT and BAT from mice housed at room temperature (RT) or 4 °C. b Immunoblot analysis of YTHDF1 and UCP1 expression in iWAT from mice treated with or without CL-316,243 (CL). c – g Y1 CTL and Y1 cKO littermates were exposed to cold conditions for 7 days. c H&E staining of iWAT. Scale bar, 50 μm. The white line indicated the average size. No adjustments. d , e Immunoblot analysis of UCP1 in iWAT d and BAT e . f , g mRNA levels of thermogenesis- and lipolysis-related genes in iWAT ( f ) and BAT ( g ) Data in f, g were presented as mean ± SEM ( n = 3 biologically indipendent mice). No adjustments. h Rectal temperature measured after exposure to cold conditions for up to 8 h, as indicated. Data were presented as mean ± SEM ( n = 3 biologically independent mice). i The O 2 consumption rate (OCR) in primary preadipocytes isolated from Y1 CTL and Y1 cKO mice determined by Seahorse. j The average basal and maximal respiration rates. Data in i , j were presented as mean ± SEM ( n = 10,000 cells exmined over 3 independent experiments). ns, not significant, * P < 0.05, ** P < 0.01, *** P < 0.001. All of the P -values are determined by unpaired two-sided t-test. Source data are provided as a Source Data file. Full size image To exclude BAT function, we surgically removed BAT. Without BAT, Ythdf1 cKO mice still had lower OCR and lower Ucp1 expression than Ythdf1 CTL mice under RT, cold, and thermoneutral conditions (Supplementary Fig. 4G-I ). Taken together, these data suggested that YTHDF1 promoted the thermogenesis of adipocytes in WAT. Transcriptome-wide identification of YTHDF1-regulated transcripts in beige adipose tissue Because YTHDF1 is an m 6 A reader protein, we performed m 6 A-seq in cold treated iWAT (Fig. 4a ). As expected, our m 6 A data revealed that the distribution of m 6 A was enriched around stop codons within transcripts (Fig. 4b ). The m 6 A peaks were characterized by the canonical RGACH motif (Fig. 4c ). YTHDF1 is known to affect mRNA translation [15] . To identify potential targets regulated by YTHDF1, we assessed changes in mRNA levels and translational efficiency by RNA-seq and ribosome profiling (Ribo‐seq) in wild-type and Ythdf1 -knockout iWAT under cold stimulation (Fig. 4a ). As expected, our data revealed a notable decrease in translational efficiency for m 6 A‐marked transcripts in Ythdf1 -knockout mice compared with that in wild-type mice (Fig. 4d ). Fig. 4: Transcriptome‐wide identification of YTHDF1‐regulated transcripts in beige adipose tissue. a Schematic description of the m 6 A-seq and RNA-seq, and Ribo-seq experiments. b Metagene plot of m 6 A peak distribution in iWAT at 4 °C. c Consensus motif of m 6 A sites in beige adipose tissue. d Violin plots showing TE changes between Ythdf1 CTL and Ythdf1 cKO mice for nonmethylated (non‐m 6 A) and methylated (m 6 A) transcripts. **** P < 0.001, Mann–Whitney test. No adjustments. e Top KEGG and GO analysis terms enriched for transcripts during beiging and downregulated translation levels. f Overlap of m 6 A targeted transcripts with translationally downregulated or upregulated genes. g Volcano plot of fold changes in translation levels from iWAT of cold-treated Y1 CTL and Y1 cKO mice. The upregulated (red) and downregulated (blue) genes are highlighted. Green dot indicates the Bmp8b gene. The other BMP genes were highlighted in yellow. Mann–Whitney test. Source data are provided as a Source Data file. Full size image To identify the functional pathways associated with YTHDF1‐targeted mRNAs, we analyzed genes that were translationally altered by Ythdf1 knockout. In total, we detected 595 downregulated genes and 560 upregulated genes from Ribo-seq data. Kyoto Encyclopedia of Genes and Genomes pathways analyses showed that the top enriched pathways of downregulated genes were associated with a series of metabolism-related pathways such as PPAR signaling pathway and fatty acid metabolism. Gene Ontology analysis revealed that cAMP catabolic process, TG homeostasis, and lipoprotein metabolic process were enriched (Fig. 4e ). The upregulated genes were enriched in nicotine addiction and cardiac muscle contraction (Supplementary Fig. 5A ). By overlapping differentially expressed genes with m 6 A-modified mRNAs, we identified 59 downregulated genes and 49 upregulated genes with m 6 A modification, which are potential YTHDF1 targets. (Fig. 4f ). Among the 59 genes, bone morphogenetic protein 8b ( Bmp8b ) was the most dramatically downregulated one (Fig. 4g ). Therefore, we picked BMP8B for further validation. YTHDF1 regulates BMP8B in an m 6 A-dependent manner The elevated expression of BMP8B in beige adipose tissue was confirmed, implying a role of BMP8B in iWAT beiging (Fig. 5a ). The Bmp8b mRNA was almost unchanged, while BMP8B protein level was downregulated in Ythdf1 cKO iWAT, implying that YTHDF1 regulated BMP8B expression at the translational level (Fig. 5b ). We analyzed BMP8B expression in BAT from Ythdf1 CTL and Ythdf1 cKO mice. Knockout of Ythdf1 did not affect BMP8B protein level and mRNA translation in BAT (Supplementary Fig. 5B–D ), suggesting that YTHDF1 regulates Bmp8b translation mainly in iWAT. Fig. 5: YTHDF1 regulates BMP8B in an m 6 A-dependent manner. a The mRNA and protein levels of BMP8B in iWAT from mice treated at RT or 4 °C. b The mRNA and protein levels of BMP8B in iWAT from Y1 CTL and Y1 cKO mice treated at 4 °C. c The mRNA level of Ythdf1 and Bmp8b in 3T3-L1 cells with or without YTHDF1 knockdown. d The protein levels of BMP8B expression in 3T3-L1 cells with or without Ythdf1 knockdown. e Polysome profiles of 3T3-L1 cells with or without YTHDF1 knockdown. f The distributions of Gapdh and Bmp8b in polysome fractions. g m 6 A peak distribution within Bmp8b transcripts. * indicates the predicted m 6 A peak. h Schematic of luciferase constructs with the predicted m 6 A sites in the CDS and 3′UTR of Bmp8b mRNA. i Luciferase activity of the Bmp8b reporter in 3T3-L1 cells with or without YTHDF1 knockdown. j Schematic of the mouse treatment regimen. k–m Mice were treated at 4 °C. k Oxygen consumption rates (OCR) of iWAT from Y1 CTL and Y1 cKO mice with or without BMP8B overexpression. Data were presented as mean ± SEM ( n = 6 biologically independent mice). **** P < 0.0001. l The expression of BMP8B and UCP1 in iWAT from Y1 CTL and Y1 cKO mice with or without BMP8B expression. m H&E staining of iWAT depots from Y1 CTL and Y1 cKO mice with or without BMP8B expression. Scale bar, 50 μm. The white line indicated the average size. No adjustments. Data in a–c, f , and i were presented as mean ± SEM ( n = 3). ns, not significant, * P < 0.05, **** P < 0.0001. All of the P -values are determined by unpaired two-sided t-test. Source data are provided as a Source Data file. Full size image To elucidate the regulatory mechanism through which YTHDF1 affected BMP8B expression, we generated Ythdf1 -knockdown pre-adipocyte 3T3-L1 cells (Fig. 5c ), which also exhibited decreased BMP8B protein level but no change in Bmp8b mRNA level (Fig. 5c, d ). Polysome profiling revealed reduced translation of Bmp8b in Ythdf1 ‐silenced cells (Fig. 5e, f ). Knockdown of YTHDF2 or YTHDF3 did not affect BMP8B expression (Supplementary Fig. 5E, F ), implying that BMP8B expression is specifically regulated by YTHDF1. Three m 6 A peaks were identified in the coding sequence (CDS) and 3’ untranslated region (UTR) of Bmp8b mRNA (nt 683–1282, 1391–1840, and 2314–2766 in the transcript ENSMUSG00000002384; Fig. 5g ). To investigate the regulation of BMP8B by YTHDF1 through m 6 A, we cloned each of the m 6 A peaks into a luciferase reporter (Fig. 5h ). Knockdown of Ythdf1 decreased Bmp8b −3’UTR-1 luciferase activity but not Bmp8b -CDS or Bmp8b −3’UTR-2 luciferase activity (Fig. 5i ), suggesting that YTHDF1 mediated the translation of the Bmp8b 3’UTR. The binding of YTHDF1 with Bmp8b mRNA was confirmed by RIP-qPCR analysis (Supplementary Fig. 5G ). Collectively, these findings suggested that the translation of Bmp8b was directly regulated by YTHDF1. To clarify the functional relationship between BMP8B and YTHDF1, we performed rescue experiments by expressing FLAG-tagged BMP8B in Ythdf1 -depleted iWAT using an AAV system (Fig. 5j ). Overexpression of BMP8B largely reversed the impaired beiging, changes in UCP1 expression, and OCR elicited by Ythdf1 deletion (Fig. 5k–m ). These results indicated that BMP8B was a key effector promoting WAT beiging downstream of YTHDF1. WAT-specific YTHDF1 overexpression promotes beiging We hypothesized that WAT-specific YTHDF1 overexpression may promote the beiging process and ameliorate HFD-induced obesity. Direct unilateral injection of AAVs expressing YTHDF1 (Y1 OE ) or yellow fluorescent protein (YFP) (Y1 CTL ) into the inguinal fat pads of mice was performed. All mice in this cohort were housed in individual cages at room temperature to reduce variability in the individual degree of WAT beiging. Mice were sacrificed after 3 weeks of recovery from surgery (Fig. 6a ). Our findings showed that the expression of UCP1 and BMP8B was evaluated in Y1 OE side than Y1 CTL side, with a dramatical increase in YTHDF1 overexpression (Fig. 6b ). The mRNA levels of thermogenesis- and lipolysis-related genes were elevated (Fig. 6c ). We observed an increase in iWAT beiging in Y1 OE fat pads (Fig. 6d ). To achieve adipocyte-specific expression, we used adiponectin-promoter to drive YTHDF1 expression and got similar results (Supplementary Fig. 6A, B ). Fig. 6: WAT-specific YTHDF1 overexpression promotes beiging. a Schematic of the mouse treatment regimen. b Immunoblot analysis of YTHDF1, UCP1 and BMP8B in iWAT. c mRNA levels of thermogenesis-related genes. Data were presented as mean ± SEM ( n = 4). ns, not significant, * P < 0. 05. d H&E staining of iWAT. Scale bar, 50 μm. The white line indicated the average size. No adjustments. e Schematic of the mouse treatment regimen. f Rectal temperature of Y1 CTL and Y1 OE littermates. t-test. g The OCR of iWAT from CTL and OE mice. f , g Data were presented as mean ± SEM ( n = 6). ** P < 0.01, *** P < 0.001. h The OCR in primary preadipocytes isolated from CTL and OE mice determined by Seahorse. i The average basal and maximal respiration rates in primary preadipocytes. Data in h, i were presented as mean ± SEM ( n = 10,000 cells exmined over 3 independent experiments). * P < 0. 05, ** P < 0.01. All of the P -values are determined by unpaired two-sided t-test. Source data are provided as a Source Data file. Full size image In another group, bilateral injection of YTHDF1- or YFP-AAV into the inguinal fat pads of mice was performed (Fig. 6e ). The rectal temperature, OCR, Ucp1 expression, and lipid droplets in iWAT of Y1 OE mice were dramatically increased under cold, RT, thermoneutral condition, and NE stimulation (Fig. 6f, g and Supplementary Fig. 6C–E ), supporting the enhanced thermogenic capacity. The OCR of preadipocytes isolated from Y1 OE mice was dramatically increased (Fig. 6h ). Overall, these findings indicated that overexpression of YTHDF1 in iWAT caused spontaneous WAT beiging and adipocyte thermogenesis. WAT-specific YTHDF1 overexpression ameliorates HFD-induced obesity To explore whether YTHDF1 overexpression affects obesity, direct bilateral injection of YTHDF1- or YFP-AAV into the inguinal fat pads of mice was performed, followed by HFD feeding for 8 weeks after 2 weeks of CD feeding (Fig. 7a ). As expected, YTHDF1 expression alleviated HFD-induced obesity (Fig. 7b, c ). A reduction in the weight of adipose tissue was observed in YTHDF1 expressing mice, resulting in smaller, multilocular adipocytes containing multiple lipid droplets (Fig. 7d, e ). Metabolic cage experiments demonstrated that overexpression of YTHDF1 increased oxygen consumption, carbon dioxide generation, and energy heat generation during both light and dark cycles (Fig. 7f–h ). The core temperature was much higher in YTHDF1-expressing mice (Fig. 7i ). YTHDF1-expressing mice showed blunting of HFD-induced increases in TG, CHO, and LDL levels (Fig. 7j ). Moreover, GTTs and ITTs demonstrated that glucose tolerance and insulin sensitivity were improved in YTHDF1-expressing mice (Fig. 7k, l ). Collectively, these results demonstrated that WAT-specific YTHDF1 overexpression protected against HFD-induced obesity and metabolic disorders. Fig. 7: WAT-specific YTHDF1 overexpression ameliorates HFD-induced obesity. a Schematic of the mouse treatment regimen. b – l The AAV-CTL (CTL) and AAV-Y1 (OE) littermates were fed with HFD. b Gross view of CTL and OE mice. Scale bar, 0.5 cm. c Body weights of CTL and OE mice. d Weights and gross view of iWAT, BAT, and eWAT from AAV-CTL and AAV-Y1 mice. Scale bar, 0.5 cm. e H&E staining of adipose tissue. Scale bar, 50 μm. The white line indicated the average size. f – h O 2 consumption f , CO 2 generation g , and energy heat generation h of CTL and OE mice. White and gray areas in the graphs indicate day and night, respectively. i Rectal temperature in CTL and OE mice. j Serum concentrations of TG, CHO, LDL, and HDL in CTL and OE mice. k , l Glucose tolerance k and insulin tolerance ( l ) of CTL and OE mice. Data in c – l were presented as mean ± SEM ( n = 4 biologically independent mice). ns, not significant, * P < 0. 05, ** P < 0.01, *** P < 0.001, **** P < 0.0001, two-sided t-test. Source data are provided as a Source Data file. Full size image The m 6 A “writer” METTL3 promotes while the m 6 A “eraser” FTO inhibits thermogenesis of adipocytes [20] , [21] , [22] . In this study, we discovered that YTHDF1, an m 6 A “reader” protein, contributed to adipose tissue thermogenesis and systemic metabolism. The expression of YTHDF1, rather than other YTH family members, was reduced in obese mice and upregulated in beiging adipose tissue. Ythdf1 cKO mice gained more weight and showed aggravated insulin resistance and glucose intolerance after consumption of an HFD. By contrast, WAT-specific YTHDF1 overexpression tempered obesity-related symptoms. Moreover, YTHDF1 directly regulated the expression of BMP8B, an important stimulator of adipose tissue thermogenesis. Together, these findings demonstrated that YTHDF1 played important roles in promoting beiging and antagonizing HFD-induced obesity (Supplementary Fig. 7 ). Both beige and brown adipose tissue can be activated to produce heat and take UCP1 as the main marker gene. However, the distinct feature of beige adipocytes, which distinguishes them from brown adipocytes, is their inducible and reversible thermogenic capacity in response to environmental stimuli. Emerging evidence suggests that an alternative thermogenic pathway may exist in beige fat and could contribute to the regulation of systemic energy expenditure and glucose homeostasis [7] . Intriguingly, studies showed that the metabolically active cells are mostly beige adipocytes in humans [29] , [30] . Gene expression analyses of multiple human fat depots suggest that the majority of UCP1 + fat cells in humans show beige fat characteristics instead of brown [30] , implying that beige adipocytes play an essential role in thermogenesis. Interestingly, YTHDF1 was shown to have different regulatory effects on UCP1 expression in various adipose tissues. Under cold stimulation, or HFD feeding, adipocyte-specific deletion of Ythdf1 slightly affected UCP1 expression in BAT, but dramatically downregulated UCP1 in iWAT. This may be attributed to the fact that beige adipose tissue exhibits a more rapid response to stimulation, whereas BAT expresses constitutively high levels of UCP1. These findings proved that YTHDF1 is indispensable for beige adipose tissue, indicating its potential function in regulating systemic metabolism. Therefore, we used AAV to inject iWAT in situ for Ythdf1 overexpression. Mice with Ythdf1 overexpression in iWAT showed significant alleviation of obesity-related symptoms, including glucose intolerance, insulin resistance, and TG synthesis. These findings demonstrated that YTHDF1 specifically controlled the beiging of iWAT to regulate systemic metabolism. As an m 6 A reader protein, YTHDF1 has been reported to enhance the translation of m 6 A-modified mRNAs [15] . Consistent with this, our data revealed a notable decrease in translational efficiency for m 6 A‐marked transcripts in Ythdf1 -knockout mice compared with that in wild-type mice (Fig. 4d ), suggesting that the effect of YTHDF1 on the translation of m 6 A-modified transcripts might be general for most m 6 A genes in adipocytes. Of note, not all m 6 A-modified mRNAs are YTHDF1 targets [15] , while some m 6 A-modified mRNAs are bound by YTHDF2. That is, YTHDF1 only regulates a group of m 6 A-modified mRNAs. We observed decreased Leptin mRNA level in Ythdf1 -KO iWAT (Supplementary Fig. 4E ). Leptin is hypothesized to function as a negative feedback signal in the regulation of energy balance. It activates lipolysis and promote thermogenesis of adipose tissue [31] , [32] . Downregulation of Leptin mRNA might reflect the reduced thermogenesis in Ythdf1 -KO iWAT. However, Leptin is not among the YTHDF1-regulated transcripts (Fig. 4g ). That is, the translation of Leptin is not regulated by YTHDF1. Downregulation of Leptin might be an indirect effect of Ythdf1 -KO. The regulation and function of Leptin in YTHDF1-promoted thermogenesis needs further investigation. Bmp8b shows dramatical alteration after YTHDF1 knockout. Our data showed that YTHDF1 promotes Bmp8b translation mainly in iWAT, which could be explained by the finding that the percentage of m 6 A-modified Bmp8b mRNA is much lower in BAT than iWAT (Supplementary Fig. 5H ). The detailed mechanism needs further investigation. BMP8B is an important ligand regulating adipose tissue thermogenesis and energy balance [33] . Autocrine signaling by BMP8B produced by beige/brown adipocytes enhance the energy dissipation of the cells [34] . Furthermore, adipocyte-specific Bmp8b overexpression enhances adipose tissue browning and thermogenesis [33] , [34] . Consistent with these reports, BMP8B expression was increased after cold stimulation. Importantly, BMP8B can rescue Ythdf1 -deletion-induced impaired thermogenesis and beiging. Of note, we used the CDS region of Bmp8b for overexpression, which does not have m 6 A site and cannot be regulated by YTHDF1. Therefore, in some specific Ythdf1 cKO + BMP8B mice, the expression of BMP8B was much higher than Ythdf1 CTL mice, which induces higher UCP1 expression and thermogenesis. BMP8B acts as a pan-BMP/transforming growth factor β-receptor ligand and activates SMADs to regulate transcription [35] , [36] . BMP8B stimulation has also been demonstrated to activate SMAD1/5/8 in brown and beige adipocytes [33] . We also observed altered transcription in Ythdf1 -KO tissue, which may be a secondary effect regulated by BMP8B/SMAD signaling. Thus, YTHDF1 may have applications in therapeutic strategies for the management of obesity-associated metabolic diseases. Ethics statement All animal studies were performed in compliance with the Guide for the Care and Use of Laboratory Animals by the Medical Experimental Animal Care Commission of Zhejiang University. All animal studies used the protocol that has been approved by the Medical Experimental Animal Care Commission of Zhejiang University (ZJU20220512). Mouse experiments Mice were maintained and bred in specific pathogen-free conditions at the Animal Center of Zhejiang University. All animal studies were performed in compliance with the Guide for the Care and Use of Laboratory Animals by the Medical Experimental Animal Care Commission of Zhejiang University. Only adult male mice were used in our experiments. For each experiment, about 3–6 mice were used for each group. Randomization and blinding were used for animal studies. All mice were housed in a pathogen-free and climate-controlled environment (22–25 °C, 40–60% humidity) with a 12-h light–dark cycle that provided free access to food and water unless stated otherwise. Conditional Ythdf1 KO allele ( Ythdf1 CTL ) was generated by Cyagen Biosciences (China). The fourth exon of Ythdf1 was targeted with flanking LoxP sites. AdipoQ-Cre mice were obtained from the Jackson Laboratory. All of the primers for PCR genotyping were listed in Supplementary Table1. For obese mice model, C57BL/6 J male mice at 8–10-week-old were fed with HFD (60% fat as kcal, D12492, ResearchDiet Inc, New Brunswick, NJ) for 8–12 weeks as indicated in Figures. Chow diet (10% fat as kcal, D12450J, ResearchDiet Inc) was used as control. For cold exposure, mice were individually housed in plastic cages at 4 °C for 7 days. For thermoneutral condition, mice were individually housed in plastic cages at 29 °C. Mice were intraperitoneally injected with CL316,243(Sigma) at 1 mg/kg/day for seven consecutive days. To exclude the BAT function, interscapular BAT was surgically removed [37] , [38] . The OCR of adipose tissues was performed using Clark-type oxygen electrodes (Strathkelvin Instruments) [39] . For histology analysis, adipose tissues were rinsed with DPBS and fixed in 10% formalin. Hematoxylin and eosin (H&E) staining and immunohistochemistry were performed. Cells and reagents 3T3-L1 pre-adipocytes (CL-173) and HEK293T cells (CRL-3216) are obtained from ATCC and cultured in DMEM medium (HyClone) supplemented with 10% fetal bovine serum (Thermo Fisher Scientific). The primary preadipocytes were digested in Dispase II (Sigma-Aldrich) and cultured in DMEM/F12 medium (Gibco) [40] . The seahorse assay was performed using Seahorse XF96 Analyzer (Agilent). Plasmids construction To construct shRNA for YTHDF1-shRNA virus, shRNA oligos of YTHDF1 were cloned to the lentiviral vector pLKO.1. Transgenes encoding YFP or YTHDF1 were inserted into the multiple cloning sites of rAAV2 vector. To achieve adipose tissue-specific expression, the promoter in the vector was replaced with AdipoQ promoter. 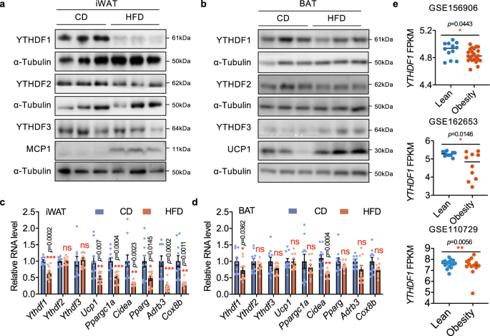Fig. 1: Adipose YTHDF1 expression is reduced in obesity. a,bImmunoblot analysis of YTH family proteins in iWATaand BATbof mice fed with CD or HFD for 12 weeks.c, dmRNA levels ofYthfamily genes and thermogenesis-related genes in iWATcand BATdof CD- and HFD-fed mice. Data were presented as mean ± SEM (n= 10). ns, not significant, *P< 0.05, **P< 0.01, ***P< 0.001, two-sided t-test.eExpression ofYTHDF1in human white adipose tissues from GSE156906 (nLean= 14,nObesity= 27, two-sided t-test), GSE162653 (n= 10, two-sided t-test), and GSE110729 (nLean= 15,nObesity= 13, F-test). Source data are provided as a Source Data file. The oligos for shRNA construction are listed in Supplementary Table 1. RNA isolation and quantitative RT-PCR Total RNA was isolated from various adipose tissues of mice or cells using TRIzol reagent (Life Technologies). Reverse transcription of RNA sample with M-MLV reagent (Takara) using random primers. Real-time PCR was performed using the SYBR Green I master mix (Takara) on a Light Cycler 480 real-time PCR system (Roche). Relative gene expression was normalized for the ACTB or GAPDH reference gene and was calculated using the 2(−ΔΔCT) method. 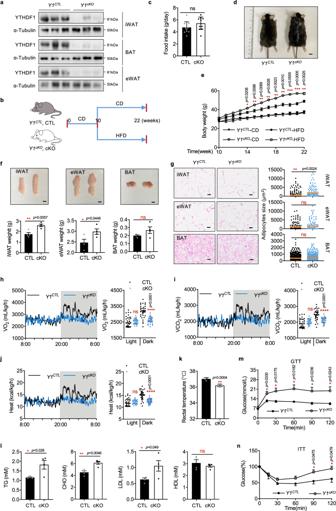Fig. 2: Adipocyte-specific knockout ofYthdf1predisposes mice to HFD-induced obesity. aImmunoblotting of adipose tissues fromY1CTLandY1cKOmice.bSchematic of the mouse treatment regimen.c–nTheY1CTLandY1cKOlittermates were fed with HFD.cDaily food intake byY1CTLandY1cKOmice.dGross view ofY1CTLandY1cKOmice. Scale bar, 0.5 cm.eBody weights ofY1CTLandY1cKOmice.fGross view and weights of iWAT, eWAT, and BAT fromY1CTLandY1cKOmice. Scale bar, 0.5 cm.gH&E staining of iWAT eWAT, and BAT fromY1CTLandY1cKOmice. Scale bar, 50 μm. The red line indicated the average size. No adjustments.h–jO2consumptionh, CO2generationi, and energy heat generationjofY1CTLandY1cKOmice. White and gray areas in the graphs indicate day and night, respectively.kRectal temperature inY1CTLandY1cKOmice.lSerum concentrations of TG, CHO, LDL, and HDL inY1CTLandY1cKOmice fed with HFD.m,nglucose tolerancemand Insulin tolerancenfed with HFD. Data inc,e–nwere presented as mean ± SEM (n= 4 biologically independent mice). ns, not significant, *P< 0.05, **P< 0.01, ****P< 0.0001, two-sided t-test. Source data are provided as a Source Data file. RT-qPCR primers are listed in Supplementary Table 2. Immunoblotting Cells or adipose tissues were lysed in RIPA lysis buffer (Beyotime, China). Total protein under denaturing conditions was separated by sodium dodecyl sulfate-polyacrylamide gel (SDS-PAGE) and transferred to PVDF membranes (Millipore). Membranes were blocked and incubated with primary antibodies, followed by incubation with the secondary antibody and chemiluminescent detection system (Bio-Rad). Anti-YTHDF1 (Proteintech, 17479-1-AP), Anti-YTHDF2 (Proteintech, 24744-1-AP), Anti-YTHDF3 (Proteintech, 25537-1-AP), Anti-UCP1 (Proteintech, 23673-−1-AP), Anti-MCP1 (Abcam, ab214819), Anti-BMP8B (Shanghai Huzhen, HZ-12837R) were used for immunoblotting at 1:1000 dilution. Anti-Alpha-Tubulin (Abclonal, A6830) and anti-ACTB (Proteintech, 66009-1-Ig) were used for immunoblotting at 1:3000 dilution. Polysome Profiling Cells or tissues were lysed in polysome lysis buffer (10 mM HEPES, pH 7.4, 100 mM KCl, 5 mM MgCl 2 , 100 μg/ml CHX, 5 mM DTT, and 1% Triton X‐100) and centrifuged. The supernatant was centrifuged in gradient sucrose (Beckman, rotor SW41Ti), fractioned (BioCamp), and collected (FC203B, Gilson). Total RNA from the indicated fractions were isolated by TRIzol reagent for RT-qPCR analysis [41] . Virus packaging The lentivirus was packaged in HEK293T cells with helper vector pMD2G and psPAX2 by transfecting cells with indicated constructs. The AAV was packaged with pAAV-RC2 and pHelper in AAV293 cells. rAAV injection to inguinal WAT A total of 6-week-old mice were anesthetized with 2% isoflurane in O 2 . After anesthesia was fully induced, mice were injected with rAAV (1.0 × 10 12 vg per 20 μl phosphate buffered saline) with a 0.3 cc, 30 G insulin syringe [42] . Finally, the wound was closed with 4-0 PDS II FS-2 suture. Metabolic analysis Body weight and food intake were measured weekly. For GTT, mice were intraperitoneally injected of D-glucose (2 g/kg body weight, 1 g/kg body weight for obese mice) after overnight starvation. For ITT, mice were intraperitoneally injected with insulin (0.7 U/kg body weight, 1.5 U/kg body weight for obese mice) after 5 hr fasting. Serum glucose levels were determined in tail blood samples at 0, 15, 30, 60, 90, and 120 min after glucose or insulin injection using a glucometer (Accu-Chek, Roche). Core body temperature was measured intra-rectally at around 4 p.m. The energy expenditure, including O 2 consumption, CO 2 generation, and energy heat generation, were monitored using Promethion High-Definition Behavioral Phenotyping System for Mice (Sable Systems International). Biochemical analysis of plasma Blood samples were obtained from cardiac puncture, and plasma was collected after centrifugation for 15 min at 3000 rpm at 4 °C. Total cholesterol, triglyceride, low-density lipoprotein cholesterol and high-density lipoprotein cholesterol were measured by using the assay kits were from HaoKe Biotech Co., Ltd. (Shanghai, China). RNA-seq The polyadenylated RNA was enriched from total RNA using the Dynabeads Oligo(dT)25 (Invitrogen, USA) and fragmented into ~100-nucleotide-long fragments using RNA fragmentation reagent (Ambion, AM8740). Fragmented RNA samples were used for library construction and high‐throughput sequencing. m 6 A-seq Fragmented mRNA was incubated with m 6 A antibody-coated beads for 6 h at 4 °C. The immunoprecipitation complex was digested with Proteinase K at 55 °C for 1 h. RNA was then extracted using TRIzol reagent and used for library construction. Ribo-seq iWAT tissue was treated with polysome lysis buffer. After centrifugation, the supernatant was digested with E. coli RNase I (Ambion) for 1 h. Ribosome-protected fragments were collected by ultracentrifugation. RNA was extracted using TRIzol reagent. The library was constructed with small RNA library construction kit (NEB) [41] . Statistical analysis Illumina Casava1.7 software used for basecalling. Sequenced reads were trimmed for adaptor sequence, and masked for low-complexity or low-quality sequence, then mapped to mm8 whole genome using Hisat2 v2.2.1 [41] . Statistical analysis was performed using GraphPad Prism 8 software (GraphPad Software, Inc.). Data were presented as mean ± standard errors of the means (SEM). P values were calculated using a two‐tailed t‐test unless stated otherwise. Asterisks denote statistical significance (* P < 0.05; ** P < 0.01; *** P < 0.001; **** P < 0.0001). 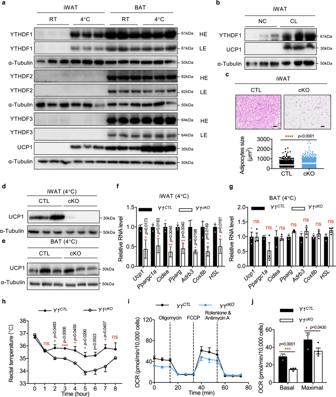Fig. 3: Adipocyte-specific knockout ofYthdf1inhibits beiging of iWAT. aImmunoblot analysis of YTH family proteins expression in iWAT and BAT from mice housed at room temperature (RT) or 4 °C.bImmunoblot analysis of YTHDF1 and UCP1 expression in iWAT from mice treated with or without CL-316,243 (CL).c–gY1CTLandY1cKOlittermates were exposed to cold conditions for 7 days.cH&E staining of iWAT. Scale bar, 50 μm. The white line indicated the average size. No adjustments.d,eImmunoblot analysis of UCP1 in iWATdand BATe.f,gmRNA levels of thermogenesis- and lipolysis-related genes in iWAT (f) and BAT (g) Data inf, gwere presented as mean ± SEM (n= 3 biologically indipendent mice). No adjustments.hRectal temperature measured after exposure to cold conditions for up to 8 h, as indicated. Data were presented as mean ± SEM (n= 3 biologically independent mice).iThe O2consumption rate (OCR) in primary preadipocytes isolated fromY1CTLandY1cKOmice determined by Seahorse.jThe average basal and maximal respiration rates. Data ini,jwere presented as mean ± SEM(n= 10,000 cells exmined over 3 independent experiments). ns, not significant, *P< 0.05, **P< 0.01, ***P< 0.001. All of theP-values are determined by unpaired two-sided t-test. Source data are provided as a Source Data file. 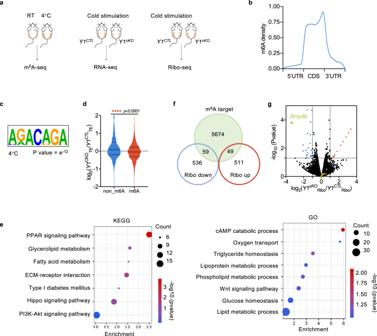Fig. 4: Transcriptome‐wide identification of YTHDF1‐regulated transcripts in beige adipose tissue. aSchematic description of the m6A-seq and RNA-seq, and Ribo-seq experiments.bMetagene plot of m6A peak distribution in iWAT at 4 °C.cConsensus motif of m6A sites in beige adipose tissue.dViolin plots showing TE changes betweenYthdf1CTLandYthdf1cKOmice for nonmethylated (non‐m6A) and methylated (m6A) transcripts. ****P< 0.001, Mann–Whitney test. No adjustments.eTop KEGG and GO analysis terms enriched for transcripts during beiging and downregulated translation levels.fOverlap of m6A targeted transcripts with translationally downregulated or upregulated genes.gVolcano plot of fold changes in translation levels from iWAT of cold-treatedY1CTLandY1cKOmice. The upregulated (red) and downregulated (blue) genes are highlighted. Green dot indicates theBmp8bgene. The other BMP genes were highlighted in yellow. Mann–Whitney test. Source data are provided as a Source Data file. 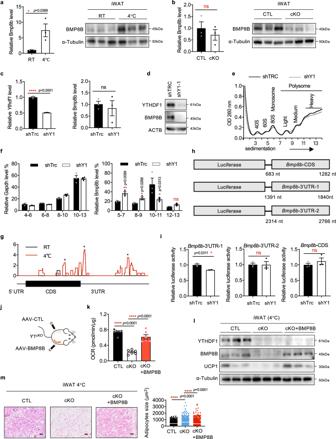Fig. 5: YTHDF1 regulates BMP8B in an m6A-dependent manner. aThe mRNA and protein levels of BMP8B in iWAT from mice treated at RT or 4 °C.bThe mRNA and protein levels of BMP8B in iWAT fromY1CTLandY1cKOmice treated at 4 °C.cThe mRNA level ofYthdf1andBmp8bin 3T3-L1 cells with or without YTHDF1 knockdown.dThe protein levels of BMP8B expression in 3T3-L1 cells with or withoutYthdf1knockdown.ePolysome profiles of 3T3-L1 cells with or without YTHDF1 knockdown.fThe distributions ofGapdhandBmp8bin polysome fractions.gm6A peak distribution withinBmp8btranscripts. * indicates the predicted m6A peak.hSchematic of luciferase constructs with the predicted m6A sites in the CDS and 3′UTR ofBmp8bmRNA.iLuciferase activity of theBmp8breporter in 3T3-L1 cells with or without YTHDF1 knockdown.jSchematic of the mouse treatment regimen.k–mMice were treated at 4 °C.kOxygen consumption rates (OCR) of iWAT fromY1CTLandY1cKOmice with or without BMP8B overexpression. Data were presented as mean ± SEM (n= 6 biologically independent mice). ****P< 0.0001.lThe expression of BMP8B and UCP1 in iWAT fromY1CTLandY1cKOmice with or without BMP8B expression.mH&E staining of iWAT depots fromY1CTLandY1cKOmice with or without BMP8B expression. Scale bar, 50 μm. The white line indicated the average size. No adjustments. Data ina–c, f, andiwere presented as mean ± SEM (n= 3). ns, not significant, *P< 0.05, ****P< 0.0001. All of theP-values are determined by unpaired two-sided t-test. Source data are provided as a Source Data file. 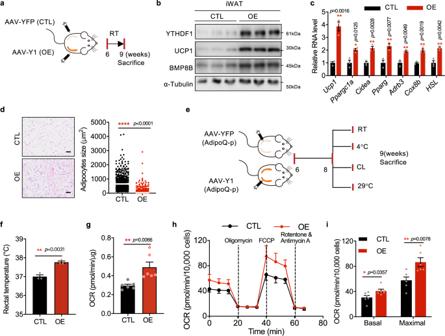Fig. 6: WAT-specific YTHDF1 overexpression promotes beiging. aSchematic of the mouse treatment regimen.bImmunoblot analysis of YTHDF1, UCP1 and BMP8B in iWAT.cmRNA levels of thermogenesis-related genes. Data were presented as mean ± SEM (n= 4). ns, not significant, *P< 0. 05.dH&E staining of iWAT. Scale bar, 50 μm. The white line indicated the average size. No adjustments.eSchematic of the mouse treatment regimen.fRectal temperature of Y1CTLand Y1OElittermates. t-test.gThe OCR of iWAT from CTL and OE mice.f,gData were presented as mean ± SEM (n= 6). **P< 0.01, ***P< 0.001.hThe OCR in primary preadipocytes isolated from CTL and OE mice determined by Seahorse.iThe average basal and maximal respiration rates in primary preadipocytes. Data inh, iwere presented as mean ± SEM (n= 10,000 cells exmined over 3 independent experiments). *P< 0. 05, **P< 0.01. All of theP-values are determined by unpaired two-sided t-test. Source data are provided as a Source Data file. 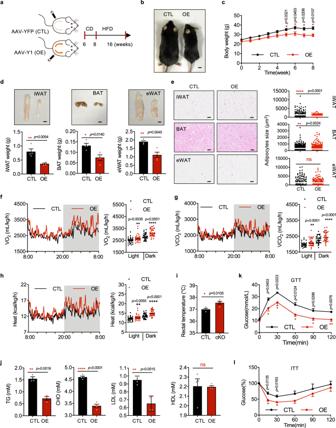Fig. 7: WAT-specific YTHDF1 overexpression ameliorates HFD-induced obesity. aSchematic of the mouse treatment regimen.b–lThe AAV-CTL (CTL) and AAV-Y1 (OE) littermates were fed with HFD.bGross view of CTL and OE mice. Scale bar, 0.5 cm.cBody weights of CTL and OE mice.dWeights and gross view of iWAT, BAT, and eWAT from AAV-CTL and AAV-Y1 mice. Scale bar, 0.5 cm.eH&E staining of adipose tissue. Scale bar, 50 μm. The white line indicated the average size.f–hO2consumptionf, CO2generationg, and energy heat generationhof CTL and OE mice. White and gray areas in the graphs indicate day and night, respectively.iRectal temperature in CTL and OE mice.jSerum concentrations of TG, CHO, LDL, and HDL in CTL and OE mice.k,lGlucose tolerancekand insulin tolerance (l) of CTL and OE mice. Data inc–lwere presented as mean ± SEM (n= 4 biologically independent mice). ns, not significant, *P< 0. 05, **P< 0.01, ***P< 0.001, ****P< 0.0001, two-sided t-test. Source data are provided as a Source Data file. Statistics and reproducibility All of the experiments had repeated at least 3 times independently with similar results. Reporting summary Further information on research design is available in the Nature Portfolio Reporting Summary linked to this article.